Length-dependent thermal conductivity in suspended single-layer graphene Graphene exhibits extraordinary electronic and mechanical properties, and extremely high thermal conductivity. Being a very stable atomically thick membrane that can be suspended between two leads, graphene provides a perfect test platform for studying thermal conductivity in two-dimensional systems, which is of primary importance for phonon transport in low-dimensional materials. Here we report experimental measurements and non-equilibrium molecular dynamics simulations of thermal conduction in suspended single-layer graphene as a function of both temperature and sample length. Interestingly and in contrast to bulk materials, at 300 K, thermal conductivity keeps increasing and remains logarithmically divergent with sample length even for sample lengths much larger than the average phonon mean free path. This result is a consequence of the two-dimensional nature of phonons in graphene, and provides fundamental understanding of thermal transport in two-dimensional materials. In bulk materials, heat conduction is governed by Fourier’s law: J =− κ ∇ T , where J is the local heat flux, ∇ T is the temperature gradient and κ is thermal conductivity, which is an intrinsic parameter of the materials and is usually size and geometry independent. Over the past 200 years, Fourier’s law has been successfully employed to describe thermal conduction in three-dimensional systems. However, with the recent availability of low-dimensional materials, it remains to verify whether thermal conductivity is still size/geometry independent. For one-dimensional (1D) lattice models [1] , [2] , [3] , [4] , [5] and quasi-1D nanostructures and polymers [6] , [7] , [8] , a length dependence of κ as~ L β ( L is sample length) has been predicted theoretically and then experimentally verified for nanotubes [9] . The same question remains open for two-dimensional (2D) systems. While logarithmic divergence of the thermal conductivity has been demonstrated numerically for 2D lattice models [2] , [3] , [10] , [11] , [12] , [13] , simulations of bi-dimensional materials such as graphene, give contradictory results, which depend on the employed simulation techniques and approximations [14] , [15] , [16] , [17] . Graphene is believed to be a perfect test bed to investigate this size effect of 2D systems owing to its novel thermal properties [18] , [19] , [20] , [22] , [24] , [25] , [26] , [27] , [28] , [29] , [30] , [31] , [32] , [33] . However, besides a recent experiment carried out on supported graphene nanoribbons [34] , in which size effect, especially the length effect, is affected by graphene–substrate interaction [35] , a compelling experimental investigation of length-dependent thermal conductivity in suspended single-layer graphene (SLG) is still missing, probably owing to the challenges in suspending this atomically thick membrane suitable for size-dependent thermal measurements. Here we report measurements of thermal conduction in suspended SLG grown by chemical vapour deposition on copper (Cu-CVD) [36] , [37] , [38] . Both the experimental and simulation results show that thermal conductivity scale with length as κ ~log L at room temperature even when L is one order of magnitude larger than the average phonon mean free path (MFP), which we think is related to the 2D nature of phonons in graphene. Possible mechanisms of this divergent behaviour are discussed. Temperature-dependent thermal conduction The experimentally measured thermal conductance σ =1/ R total and κ for all junctions are shown in Fig. 1c,d . Here κ is obtained from , in which R total is the total measured thermal resistance, R c is the thermal contact resistance and A is the unit cross-section area (we define A = w × h , where w is the width of the samples and h ≈0.34 nm is the nominal thickness of SLG). Independently on the sample length, all samples exhibit qualitatively the same behaviour as a function of the temperature: σ ( T ) increases with temperature and reaches a broad plateau. The thermal conductivity at T =300 K in our longest sample ( L =9 μm) shows a value of (1,689±100) Wm −1 K −1 ~(1,813±111) Wm −1 K −1 (see Supplementary Note 1 ; Supplementary Tables 1 and 2 for the error bars), which is comparable to the values obtained from Raman-based measurement techniques (from ~1,800 Wm −1 K −1 to ~5,300 Wm −1 K −1 , see Supplementary Note 2 ; Supplementary Table 3 ). Remarkably, our measurements show that κ increases with sample length over the entire measured temperature range. 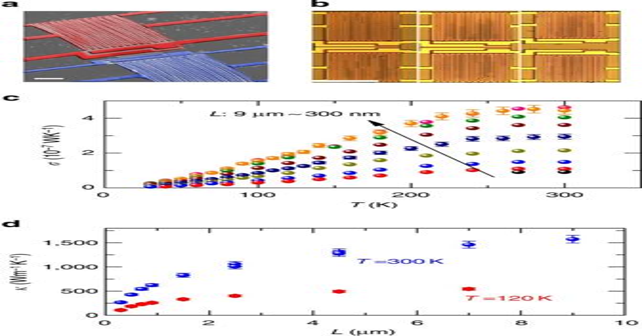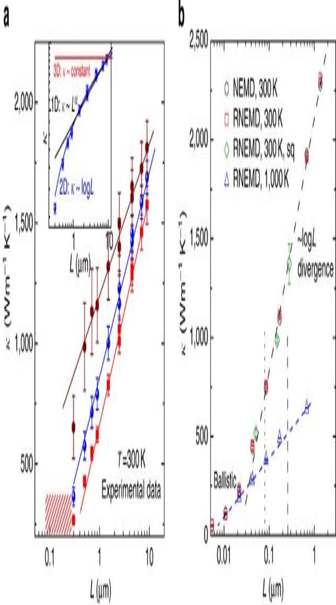Figure 3: Experimental and simulation results on length-dependent thermal conductivity. (a) Length dependence of the extracted intrinsic thermal conductivity when assumingRccontributes negligible (red squares), 5% (blue circles) and 11.5% (brown diamonds) to the total measured thermal resistance in a 9-μm-long sample. The linear solid lines are guides to the eyes. The red diagonal lines indicate the average/effective phonon mean free path (MFP), which is 240 nm and 80 nm obtained by experiment and simulation, respectively. Inset: illustration of logκ~logLscaling behaviour for one-dimensional (1D), two-dimensional (2D) and three-dimensional (3D) systems, where thermal conductivity scales as ~L0.33, ~logLand constant, respectively. Also seeSupplementary Fig. 8. (b)Thermal conductivity of graphene as a function of the distance between the hot and the cold reservoir, obtained with direct (black circles) and reverse non-equilibrium molecular dynamics (NEMD) (red squares and green diamonds) methods atT=300 K and reverse NEMD at 1,000 K (blue triangles). Results obtained with supercells with square aspect ratio (green diamonds) agree well with those obtained with elongated supercells (all others). Dashed lines indicate the logarithmic fit. The dotted and dashed vertical lines indicate the limit of the ballistic transport regime obtained by experiment and simulation, respectively. Figure 1: Thermal conduction versus temperature. (a) False-colour scanning electron microscopy image of the suspended device, which consists of two 25 × 20 μm2Pt/SiNxmembranes. The red and blue Pt coils are the heater (Rh) and sensor (Rs), which are thermally connected by suspended graphene (grey sheet in the middle). Scale bar, 5 μm. (b) SiNxmembrane-based heater structures optimized for length-dependent studies. Scale bar, 20 μm. (c) Total measured thermal conductance (σ) versus temperature. The sample with 9 μm broke when cooling below 270 K during measurements. Also seeSupplementary Fig. 7. (d) Thermal conductivity (κ) versus sample length (L) with negligible thermal contact resistanceRcatT=300 K and 120 K, respectively. Figure 1: Thermal conduction versus temperature. ( a ) False-colour scanning electron microscopy image of the suspended device, which consists of two 25 × 20 μm 2 Pt/SiN x membranes. The red and blue Pt coils are the heater ( R h ) and sensor ( R s ), which are thermally connected by suspended graphene (grey sheet in the middle). Scale bar, 5 μm. ( b ) SiN x membrane-based heater structures optimized for length-dependent studies. Scale bar, 20 μm. ( c ) Total measured thermal conductance ( σ ) versus temperature. The sample with 9 μm broke when cooling below 270 K during measurements. Also see Supplementary Fig. 7 . ( d ) Thermal conductivity ( κ ) versus sample length ( L ) with negligible thermal contact resistance R c at T =300 K and 120 K, respectively. Full size image Quasi-ballistic phonon transport in submicron samples Here plotting σ /A is more instructive than κ . In all submicron samples, the thermal conductance exhibits the same temperature dependence ( Fig. 2a ). This has important implications for the nature of 2D phonon transport. It has been reported that phonons in graphene can travel without scattering, that is, ballistic transport [34] , [39] . In clean devices, σ/A has been expected to follow Wm −2 K −1 , as shown by the black dashed curve in the same figure [34] . 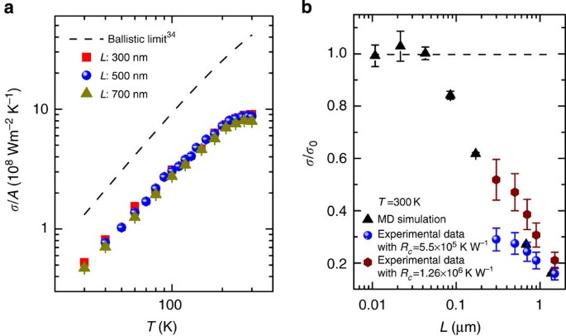Indeed, the experimentally measured values are not only length independent, but also within 39.8% of the predicted ballistic thermal conductance at T =30 K (phonons in quasi-ballistic regime at low temperature), indicating high sample quality and clean surface in the measured graphene. Figure 2: Thermal conductance in submicron devices. (a) Experimental thermal conductance per unit cross-section areaσ/Aas a function of temperature in samples withL: 300 nm–700 nm. The ballistic limit is indicated by the black dashed curve34. (b) Molecular dynamics (MD) simulation results (black triangles) of thermal conductanceσ/σ0versus sample lengthLatT=300 K. Simulation results are compared with experiments (blue circles and brown diamonds) assuming different values of thermal contact resistanceRc. The MD thermal conductance is normalized toσ0, whereσ0is the calculated thermal conductance in a sample with 5.5 nm between the hot and the cold reservoir; the experimental data are normalized to the ballistic limit shown inFig. 2aatT=300 K, that is,σ0/A=4.17 × 109Wm−2K−1. Figure 2: Thermal conductance in submicron devices. ( a ) Experimental thermal conductance per unit cross-section area σ / A as a function of temperature in samples with L : 300 nm–700 nm. The ballistic limit is indicated by the black dashed curve [34] . ( b ) Molecular dynamics (MD) simulation results (black triangles) of thermal conductance σ / σ 0 versus sample length L at T =300 K. Simulation results are compared with experiments (blue circles and brown diamonds) assuming different values of thermal contact resistance R c . The MD thermal conductance is normalized to σ 0 , where σ 0 is the calculated thermal conductance in a sample with 5.5 nm between the hot and the cold reservoir; the experimental data are normalized to the ballistic limit shown in Fig. 2a at T =300 K, that is, σ 0 / A =4.17 × 10 9 Wm −2 K −1 . Full size image Atomistic simulations provide a powerful tool for validation and interpretation of experimental measurements, with the advantage that the limit of perfectly crystalline samples can be probed. We have performed non-equilibrium molecular dynamics (NEMD) [40] simulations of heat transport in graphene at similar conditions as the experiments. We considered periodic models of defect-free, isotopically pure and suspended graphene patches with sizes between 5.5 nm and 1.4 μm, at 300 K and at 1,000 K. Our simulations show that at 300 K, the thermal conductance remains constant for a length (between the hot and the cold reservoir) up to ~80 nm ( σ / σ 0 =0.84 at ~80 nm, where σ 0 is the calculated thermal conductance in a 5.5-nm-long sample), indicating ballistic heat transport in this size range ( Fig. 2b ). Length-dependent thermal conductivity Before we discuss the length dependence of thermal transport at room temperature, we need to comment on the issue of thermal contact resistance R c , a critical parameter in thermal conductivity studies in general. Note that while achieving low values for R c with 1D nanowires and nanotubes remains difficult, the inherently larger contact area with 2D sheets makes it less challenging. Our calculations give a relatively small value of R c with values ranging from ~9.9 × 10 4 K W −1 to ~1.26 × 10 6 K W −1 , which contributes ~0.9% to ~11.5% of R total in the sample with 9 μm length (see Supplementary Note 3 ; Supplementary Table 4 ). Therefore, we plot κ versus L in Fig. 3a for different thermal contact resistance, that is, negligible R c , R c =5.5 × 10 5 K W −1 (~5% of R total in 9 μm sample), and R c =1.26 × 10 6 K W −1 (~11.5% of R total in 9 μm sample), respectively. κ increases with sample length at T =300 K. Surprisingly and in contrast with experiments on supported graphene [34] , κ does not saturate even in our longest sample with L =9 μm. More importantly, κ scales with ~log L in samples with L ≥700 nm (we do not claim the ~log L behaviour in shorter samples owing to the large effects from R c ). Such behaviour has been predicted for 2D systems and is a direct consequence of the 2D nature of phonons [2] , [3] . This anomalous length-dependent thermal conductivity should not be confused with quasi-ballistic transport discussed above, which occurs when the length of the sample is comparable to the average phonon MFP of the main heat carriers, that is, acoustic phonons in graphene. Following the parameters used by Ghosh et al. [28] , we estimate the average MFP to be around 240 nm at T =300 K. Please note that MFP is a spectral property that depends on frequency and polarization of each phonon, therefore MFP=240 nm is an average or effective MFP of all the phonons contributing to thermal conduction. Moreover, our simulation results show that the thermal conductance starts decreasing for length between 43 nm and 80 nm (triangles in Fig. 2b ) and is σ / σ 0 ~0.6 for L ~171 nm. Therefore , L >MFP holds in our shortest samples at T =300 K and κ does not saturate even when the length of the sample is >30 times larger than the average MFP. Figure 3: Experimental and simulation results on length-dependent thermal conductivity. ( a ) Length dependence of the extracted intrinsic thermal conductivity when assuming R c contributes negligible (red squares), 5% (blue circles) and 11.5% (brown diamonds) to the total measured thermal resistance in a 9-μm-long sample. The linear solid lines are guides to the eyes. The red diagonal lines indicate the average/effective phonon mean free path (MFP), which is 240 nm and 80 nm obtained by experiment and simulation, respectively. Inset: illustration of log κ ~log L scaling behaviour for one-dimensional (1D), two-dimensional (2D) and three-dimensional (3D) systems, where thermal conductivity scales as ~ L 0.33 , ~log L and constant, respectively. Also see Supplementary Fig. 8 . ( b )Thermal conductivity of graphene as a function of the distance between the hot and the cold reservoir, obtained with direct (black circles) and reverse non-equilibrium molecular dynamics (NEMD) (red squares and green diamonds) methods at T =300 K and reverse NEMD at 1,000 K (blue triangles). Results obtained with supercells with square aspect ratio (green diamonds) agree well with those obtained with elongated supercells (all others). Dashed lines indicate the logarithmic fit. The dotted and dashed vertical lines indicate the limit of the ballistic transport regime obtained by experiment and simulation, respectively. Full size image It is worth pointing out that, in contrast with 2D lattice models [10] , [13] , graphene atoms can move out of plane, giving rise to flexural acoustic (ZA) and flexural optical (ZO) modes. The role of the ZA modes of graphene in heat transport is still debated: according to lattice dynamics calculations and equilibrium molecular dynamics (MD) simulations, the ZA modes provide the fundamental scattering channels to limit κ to a finite value, unless strain is applied [16] , [17] . On the other hand calculations that take into account the deviations of phonon populations from equilibrium, through a self-consistent solution of the Peierls–Boltzmann equation, suggest that ZA modes are the main heat carriers in graphene, and show a significant size dependence of κ at the micrometre scale [41] . Here we have probed direct stationary non-equilibrium heat transport at conditions very similar to the experiments by NEMD simulations. In sharp contrast with previous equilibrium MD simulations, but in excellent agreement with experiments, we observe κ ( L )~log L both at T =300 K and at 1,000 K, for systems with size well beyond the ballistic length ( Fig. 3b ). Surprisingly, in spite of the unavoidable presence of boundary scattering at the interface with the thermal reservoirs, κ from NEMD exceeds the converged value of κ from equilibrium Green–Kubo calculations, computed with the same empirical potential, indicating that the mechanism of heat transport is substantially different at stationary non-equilibrium. We also note that different NEMD approaches, namely reverse NEMD [40] and direct NEMD [42] , give the same result at any given size. In addition for each L , κ ( L ) is not sensitive to the magnitude of the applied heat flux or temperature gradients. In our NEMD simulations, we ensured that grad( T ) is proportional to J , meaning that we do not break the linear response regime (see Supplementary Note 4 ; Supplementary Fig. 1 ). We have also carefully considered the effect of different aspect ratios of the simulation cell, probing very large systems of square aspect ratio, which give results in agreement with those obtained with elongated supercells ( Fig. 3b ), and confirm that the log( L ) divergence is not an artifact of the simulation setup. We now seek to understand the physics behind the observed length-dependent thermal conductivity. A number of theoretical and computational studies on ideal systems, such as the Fermi–Pasta–Ulam model, have demonstrated that κ in low-dimensional systems depends on system size (inset of Fig. 3a ). In fact, rigorous mathematical proof tells us that for a momentum-conserved 1D system, κ diverges with system size [1] , [2] , [3] , [4] , which has been confirmed experimentally in nanotubes [9] . On the other hand, the length dependence of 2D systems remains unresolved and a ~log L dependence has been proposed by various analytical theories [2] , [3] , [10] , [13] . Our experiment and simulation studies provide strong evidence for a ~log L behaviour in graphene, which is different from both of that in 1D and three-dimensional systems. The other possible mechanism behind the length-dependent thermal conductivity is related to the ballistic propagation of extremely long-wavelength, low-frequency acoustic phonons [29] , [43] . Nika et al. [29] emphasized the importance of low-frequency acoustic phonons in graphene. As sample size increases, more low-frequency acoustic phonons can be excited and contribute to thermal conduction, resulting in a length-dependent behaviour. The third possibility is related to the selection rules for three-phonon scattering, the phase space of which is strongly restricted by the reduced dimensionality [41] , [44] ; however, a non-logarithmic dependence of the thermal conductivity was reported when three-phonon process was considered to second order. A comparative analysis of phonon populations in MD simulations at equilibrium and non-equilibrium conditions suggests that in the latter conditions the population of out-of-plane modes is augmented, whereas in-plane modes with polarization in the direction of the heat flux propagation get slightly depopulated (see Supplementary Fig. 2 ). Such population imbalance produces the observed discrepancy between equilibrium and non-equilibrium simulations, promoting logarithmic divergence of κ at stationary non-equilibrium (see Supplementary Note 4 and Methods for further details). Our simulations therefore suggest that logarithmic divergence stems from the combination of reduced dimensionality and displacements of phonon populations at stationary non-equilibrium conditions. From experiments, it is still challenging to distinguish which transport mechanism dominates the observed length-dependent thermal conductivity. To this end, it would be constructive to show the relative contribution to thermal conductivity from phonons with different frequencies, or to study the thermal conductivity in samples with much larger size (for example, 100 μm or even millimetre), which would however require the development of new measurement techniques. In summary, we have studied thermal conductivity in suspended SLG. Thermal conductivity has been observed to increase with the length of the samples and to scale as ~log L, even when L is one order of magnitude longer than the average phonon MFP. Possible mechanisms have been discussed: MD simulations, in excellent agreement with experiments, confirm the divergence of κ and suggest that it is related to the 2D nature of phonons in graphene, and to the change of the phonon population at stationary non-equilibrium conditions. MD simulations NEMD simulations were performed using LAMMPS ( http://lammps.sandia.gov/ ). Interatomic forces were described by the Tersoff potential with a parameter set optimized for graphene [45] . Simulations employed periodic boundary conditions in the graphene plane, and each supercell was relaxed at the simulation temperature to achieve zero in-plane stress. Two different NEMD simulation methods were used, in which the thermal conductivity is calculated directly from the temperature gradient and the heat flux via Fourier’s law. The simulation supercell is divided in contiguous slabs along the direction of heat propagation (see Supplementary Fig. 3 ). Each slab contains ~440 atoms and the temperature of each slab is calculated from its average kinetic energy ( K E ) as T =2/3 K E / k B . The two methods differ as for the mechanism employed to generate a stationary heat flux. In the direct NEMD method [42] , independent Langevin thermostats were used to control the temperature of the cold and hot slabs. In the reverse non-equilibrium MD method [31] (RNEMD) the temperature gradient is imposed by swapping the velocity of the slowest molecule in the cold slab with the velocity of the fastest one in the hot slab. After a transient period, a stationary temperature gradient is established in the system due to the imposed heat flux. However, the velocity exchange disturbs the stability of the numerical integration of the equations of motion and introduces a drift in the total energy of the system. Velocities were exchanged every 200 steps (20 fs), and we used a timestep of 0.1 fs for a stable integration of the equations of motion. Each NEMD simulation ran for at least 40 million steps, and the temperature gradient and heat flux were taken as the average over the final 10 million steps. Error bars are the s.d. of the averaged data. Supplementary Fig. 4 shows the temperature profile for two supercell sizes, using both NEMD and RNEMD methods. Temperature gradients are taken as the average slope considering both sides of the simulation cell, only in the linear regions between cold and hot layers. Such temperature gradients, although larger in RNEMD simulations than in NEMD, are comparable to the ones in the experiment. Initially, the simulation cells were increased in length while keeping a constant width of ~11 nm. This procedure implies an increase in the aspect ratio of the simulation cells from a ratio of 1 for the smallest cell (4,400 atoms), up to a ratio of ~250 for the longest cell (1.1 million atoms). In order to assure that the length dependence observed in our results was not related to the increase in aspect ratio, we also performed simulations with square cells up to ~560 nm (11.5 million atoms), which are in agreement with the observed log divergence as shown in Fig. 3b . Validation tests of the simulation methods are described in Supplementary Note 4 ; Supplementary Fig. 1 . Fabrication details We employed typical prepatterned heater wires [46] , [47] (see Fig. 1a,b ) to measure thermal conductance of suspended SLG grown by Cu-CVD [36] , [38] . Our device fabrication starts with SiN x membrane-based heater structures ( Supplementary Fig. 5a ) optimized for length-dependent studies. To obtain high-quality samples, the CVD graphene was grown by re-using the copper catalyst [37] , which in general results in better transport properties. In order to decrease the thermal contact resistance, SiN x wafer and Pt prepatterned electrodes were cleaned for an extended period of time (>10 min) in O 2 plasma, followed by immediate CVD graphene transfer. This helps to clean organic residue on the Pt electrodes and create suspended chemical bonds, resulting in a further improvement of the thermal contact to graphene [48] . The graphene sheets were then patterned by standard electron beam lithography, followed by an O 2 plasma step (see Supplementary Fig. 5c ). In a second electron beam lithography step, 30 nm Cr/Au bars were deposited on both ends of the graphene stripes to ensure good thermal contact with the Pt electrodes underneath graphene (see Supplementary Fig. 5d ). After suspending graphene by wet etching, the devices were dried using a critical point dryer to avoid damage due to surface tension. It is worth noting that we do not etch away all the silicon under SiN x pad (that is, heater and sensor), but left few micrometres to few tens of micrometres-thick silicon to act as a massive heat batch and make sure that heat spreads uniformly within the SiN x pad during thermal measurements. Graphene samples were annealed for 5 h at 300 °C in flowing hydrogen (H 2 : 150 ml min −1 , Ar: 150 ml min −1 , 1 atm) to remove possible organic residues before measurements. Sample geometry The length dependence of thermal conductivity is studied by varying the channel length from 300 nm to 9 μm. Since the thermal conductivity is also weakly width ( w ) dependent when the width is larger than 1.5 μm (see Supplementary Fig. 6 ; Supplementary Note 5 ), we have kept the width fixed at 1.5 μm. We define the direction of heat flow as length, and the perpendicular direction as width. Thermal conductivity measurement The suspended graphene sheet provides a thermal path between the two SiN x membranes that are otherwise thermally and electrically isolated from each other ( Fig. 1a ). A μA-DC current combined with an AC current (100–200 nA) was applied to the heater resistor ( R h , red Pt coil in Fig. 1a ). The DC current was used to apply Joule heat in R h and to increase its temperature ( T h ) from the environment temperature, T 0 . The AC current was used to measure the resistance of R h . The Joule heating in R h gradually dissipates through the six Pt/SiN x beams and the graphene sheet, which raises the temperature ( T s ) in the sensor resistor ( R s , blue Pt coil in Fig. 1a ). In the steady state, the thermal conductance of the graphene sheet, σ G and each of the suspended Pt/SiN x beam, σ l , can be obtained from and where Δ T h and Δ T s indicate the temperature rise in the R h and R s , Q h and Q l indicate the Joule heat applied to the heater R h and the Pt leads. The temperature change in each membrane as function of applied Joule heat was kept in the linear range. The increase in temperature, Δ T h and Δ T s , was controlled to below 5 K to minimize thermal radiation between the two membranes. All measurements were performed under vacuum conditions better than 1 × 10 −6 mbar. How to cite this article: Xu, X. et al. Length-dependent thermal conductivity in suspended single-layer graphene. Nat. Commun. 5:3689 doi: 10.1038/ncomms4689 (2014).